Evolution under monogamy feminizes gene expression inDrosophila melanogaster Many genes have evolved sexually dimorphic expression as a consequence of divergent selection on males and females. However, because the sexes share a genome, the extent to which evolution can shape gene expression independently in each sex is controversial. Here, we use experimental evolution to reveal suboptimal sex-specific expression for much of the genome. By enforcing a monogamous mating system in populations of Drosophila melanogaster for over 100 generations, we eliminated major components of selection on males: female choice and male–male competition. If gene expression is subject to sexually antagonistic selection, relaxed selection on males should cause evolution towards female optima. Monogamous males and females show this pattern of feminization in both the whole-body and head transcriptomes. Genes with male-biased expression patterns evolved decreased expression under monogamy, while genes with female-biased expression evolved increased expression, relative to polygamous populations. Our results demonstrate persistent and widespread evolutionary tension between male and female adaptation. In many animal species, males greatly differ from females in morphology, physiology and behaviour. Most of these phenotypic differences are mediated by differential gene expression in the sexes [1] , which occurs for as much as 75% of the genome in Drosophila [2] . It is unclear, however, how often each sex evolves to reach its optimal pattern of gene expression ( Fig. 1a ) or if this outcome is prevented by genetic constraints ( Fig. 1b ). Such constraints would result in persistent sexually antagonistic selection on gene expression levels (that is, unresolved intralocus sexual conflict) [3] , [4] , whereby an increase in gene expression would improve the fitness of one sex but reduce the fitness of the other sex. This has been proposed by several studies [5] , [6] , [7] and, if true, could explain the higher observed rate of expression evolution in sex-biased genes [2] . Here, we investigated how pervasive such ongoing divergent selection on sex-specific gene expression is across the transcriptome. 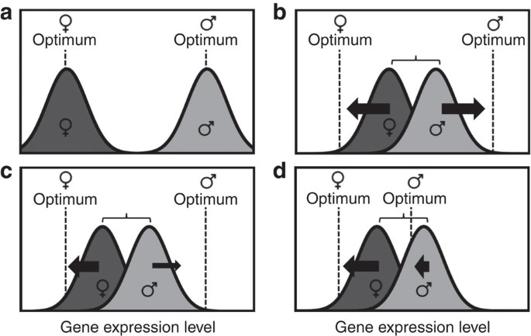Figure 1: Sexually antagonistic selection and monogamy. Levels of gene expression may experience no sexually antagonistic selection if male and female expression levels evolved to reach sex-specific optima (dashed lines) (a). Alternatively, sexually dimorphic genes may experience sexually antagonistic selection (indicated by arrows) if expression in each sex is genetically constrained (symbolized by a bracket) (b). Under monogamy, sexual selection on males may be either weakened (c) or shift the position of male optima (d), both of which favour feminization of male-biased genes (indicated by the shift in distributions). The same prediction of feminization under monogamy holds for female-biased genes. Figure 1: Sexually antagonistic selection and monogamy. Levels of gene expression may experience no sexually antagonistic selection if male and female expression levels evolved to reach sex-specific optima (dashed lines) ( a ). Alternatively, sexually dimorphic genes may experience sexually antagonistic selection (indicated by arrows) if expression in each sex is genetically constrained (symbolized by a bracket) ( b ). Under monogamy, sexual selection on males may be either weakened ( c ) or shift the position of male optima ( d ), both of which favour feminization of male-biased genes (indicated by the shift in distributions). The same prediction of feminization under monogamy holds for female-biased genes. Full size image We used experimental evolution [8] in D. melanogaster to manipulate the strength of sexual selection by imposing random monogamous mating on experimental populations [9] . This evolutionary regime eliminated major components of selection on males, including precopulatory male–male competition, female choice and sperm competition. We then contrasted the evolution of gene expression in these monogamous populations with polygamous control populations derived from the same ancestral (naturally polygamous) population [10] . If sexually antagonistic selection on gene expression is pervasive, relaxed sexual selection should cause expression patterns to evolve towards female optima, because the overall strength of selection on males is reduced ( Fig. 1c ). Furthermore, the optimal value of male expression may shift towards that of females, for example, because conflict between the sexes over mating is eliminated ( Fig. 1d ). Therefore, genes with expression levels subject to sexually antagonistic selection are expected to become feminized: male-biased genes should decline in expression in both sexes while female-biased genes should increase in expression. Consistent with this prediction, we see feminization in both the whole-body and head transcriptomes of males and females from monogamous populations. Our results thus provide experimental evidence that widespread genetic constraints impede the evolution of patterns of gene expression optimized for male and female performance. Experimental evolution We established three populations of D. melanogaster maintained under strict monogamy and three populations maintained under polygamy. In monogamous populations, individual males and females were randomly paired for mating. In polygamous populations, groups of five males and five females were placed together for mating, allowing both male–male competition and female choice. Other aspects of the experimental evolution regimes, including the number of individuals in each population and the female egg-laying and egg-to-adult development environments, were identical between selection regimes. Feminization of the transcriptome After 65 generations of evolution under the monogamous and polygamous regimes, transcriptional profiles of whole virgin males and females from all populations were obtained with NimbleGen microarrays. To compare the level of expression of male- and female-biased genes, we obtained estimates of the degree of sex-biased gene expression from the fly sex bias database, SEBIDA [11] , which classified 4,305 (35%) of the 12,301 genes as female-biased and 3,118 (25%) as male-biased. The monogamous populations exhibited a striking pattern of transcriptional feminization, consistent with the hypothesis that sexual selection is responsible for a large proportion of conflicts over sex-specific gene expression. The average level of expression of female-biased genes was 18% higher in monogamous than polygamous females, while there was an opposite effect for male-biased genes, whose levels of expression was on average 24% lower ( Fig. 2a ). This pattern of feminization was also present in males. The level of expression of female-biased genes was 7% higher in monogamous males than polygamous males while male-biased gene expression was reduced by 14% ( Fig. 2b ). There was on average no change in the level of expression of genes classified as sex-unbiased ( n =4,633) between the monogamous and polygamous selection regimes ( Fig. 2a,b ). 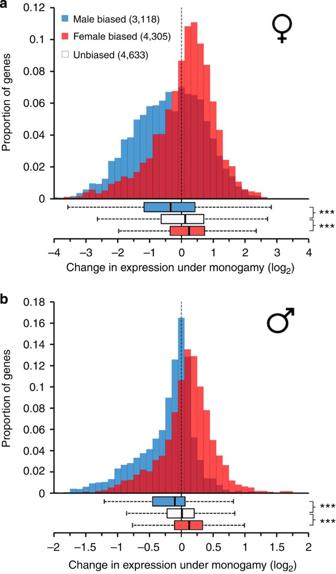Figure 2: Evolution of gene expression under monogamy in whole flies. In both the female (a) and male (b) whole-fly transcriptomes, a pattern of feminization was observed after 65 generations of evolution under monogamy. Female-biased genes (n=4,305, red ina,b) showed increased expression (relative to unbiased genes) under monogamy in both females (P<0.001) and males (P<0.001). Male-biased genes (n=3,118, blue ina,b) exhibited decreased expression (relative to unbiased genes) under monogamy in both females (P<0.001) and males (P<0.001). Genes with unbiased expression (n=4,633), depicted only in the boxplots, did not show a change significantly different than 0 under monogamy (P=0.75 for females andP=0.12 for males). Whiskers extend to 1.5 × the interquartile range, two-sample independentt-tests, ***P<0.001. Figure 2: Evolution of gene expression under monogamy in whole flies. In both the female ( a ) and male ( b ) whole-fly transcriptomes, a pattern of feminization was observed after 65 generations of evolution under monogamy. Female-biased genes ( n =4,305, red in a , b ) showed increased expression (relative to unbiased genes) under monogamy in both females ( P <0.001) and males ( P <0.001). Male-biased genes ( n =3,118, blue in a , b ) exhibited decreased expression (relative to unbiased genes) under monogamy in both females ( P <0.001) and males ( P <0.001). Genes with unbiased expression ( n =4,633), depicted only in the boxplots, did not show a change significantly different than 0 under monogamy ( P =0.75 for females and P =0.12 for males). Whiskers extend to 1.5 × the interquartile range, two-sample independent t -tests, *** P <0.001. Full size image To rule out the hypothesis that this pattern of feminization could be driven solely by changes in the size of sex-limited tissue (testes, accessory glands, ovaries and spermathecae) over the 65 generations of selection, we first conducted an analysis considering only sex-biased genes not expressed in any of the sex-limited tissues (335 genes, identified by the FlyAtlas project [12] ). This highly restricted set of genes exhibited a similar, although weaker, pattern of feminization in males as well as females ( Fig. 3a,b ). 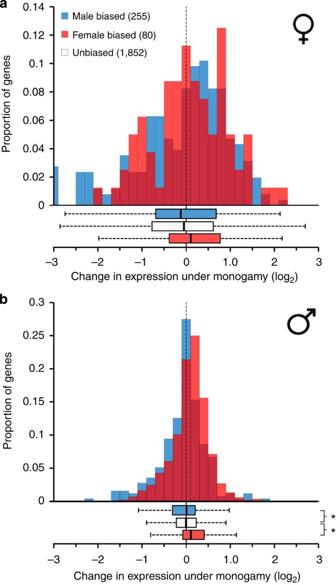Figure 3: Evolution of gene expression under monogamy for sex-biased genes that are not expressed in sex-limited tissues. The overall pattern of feminization is still observed under monogamy when considering only a strict list of sex-biased genes with no expression in the ovary, testis, accessory gland and spermatheca. In monogamous females (a), female-biased genes (n=80, red ina,b) show 7% higher expression than in polygamous females and male-biased genes (n=255, blue ina,b) show 6% lower expression, but these differences are not significantly different from unbiased gene change (P=0.05 andP=0.97, respectively). In monogamous males (b), female-biased genes show 9% higher expression while male-biased genes show 5% lower expression (P=0.02 andP=0.04, respectively). Whiskers extend to 1.5 × the interquartile range, two-sample independentt-tests, *P<0.05. Figure 3: Evolution of gene expression under monogamy for sex-biased genes that are not expressed in sex-limited tissues. The overall pattern of feminization is still observed under monogamy when considering only a strict list of sex-biased genes with no expression in the ovary, testis, accessory gland and spermatheca. In monogamous females ( a ), female-biased genes ( n =80, red in a , b ) show 7% higher expression than in polygamous females and male-biased genes ( n =255, blue in a , b ) show 6% lower expression, but these differences are not significantly different from unbiased gene change ( P =0.05 and P =0.97, respectively). In monogamous males ( b ), female-biased genes show 9% higher expression while male-biased genes show 5% lower expression ( P =0.02 and P =0.04, respectively). Whiskers extend to 1.5 × the interquartile range, two-sample independent t -tests, * P <0.05. Full size image We next used RNA-Seq to quantify expression in the heads of flies from our evolved populations after 52 more generations of experimental evolution (117 generations total). Profiling fly heads allowed us to focus on a tissue present in both sexes that still exhibits substantial sexually dimorphic gene expression [13] , [14] and also contains the brain, ultimately responsible for sexual behaviour [15] , [16] . Data from the modENCODE [17] project allowed us to identify genes with sex-biased expression in fly heads (423 male-biased genes and 46 female-biased genes with a 10% false discovery rate). These genes showed the same pattern of transcriptional feminization as in the whole-body transcriptome. In monogamous female heads, female-biased genes were expressed on average 13% higher than in polygamous female heads while expression of male-biased genes was reduced by 14% ( Fig. 4a ). Similarly, in monogamous male heads, female-biased genes were expressed 4% higher on average than in polygamous male heads, but this difference was not significant. Monogamous males also showed significantly reduced expression of male-biased genes (2% on average) relative to polygamous males ( Fig. 4b ). Finally, genes with unbiased expression ( n =4,755) again showed no average change in expression between monogamy and polygamy in either males or females ( Fig. 4a,b ). 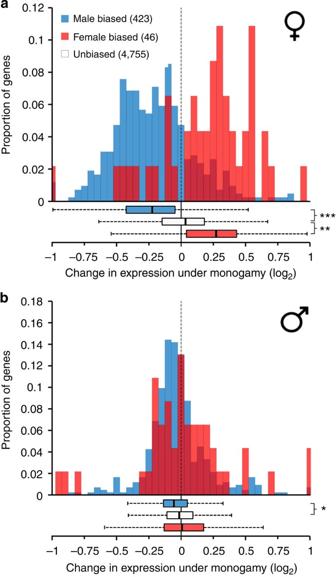Figure 4: Evolution of gene expression under monogamy in fly heads. In female (a) and male (b) fly heads, transcriptional feminization was observed after 117 generations of evolution under monogamy. Female-biased genes (n=46, red ina,b) were more highly expressed in monogamous females (P<0.01) and shift non-significantly in the same direction for males (P=0.48). Male-biased genes (n=423, blue ina,b) showed reduced expression under monogamy in both females (P<0.001) and males (P=0.02). Genes with unbiased expression (n=4,755), depicted only in the boxplots, did not show a change significantly different than 0 under monogamy (P=0.60 for females andP=0.30 for males). Whiskers extend to 1.5 × the interquartile range, two-sample independentt-tests, ***P<0.001, **P<0.01, *P<0.05. Figure 4: Evolution of gene expression under monogamy in fly heads. In female ( a ) and male ( b ) fly heads, transcriptional feminization was observed after 117 generations of evolution under monogamy. Female-biased genes ( n =46, red in a , b ) were more highly expressed in monogamous females ( P <0.01) and shift non-significantly in the same direction for males ( P =0.48). Male-biased genes ( n =423, blue in a , b ) showed reduced expression under monogamy in both females ( P <0.001) and males ( P =0.02). Genes with unbiased expression ( n =4,755), depicted only in the boxplots, did not show a change significantly different than 0 under monogamy ( P =0.60 for females and P =0.30 for males). Whiskers extend to 1.5 × the interquartile range, two-sample independent t -tests, *** P <0.001, ** P <0.01, * P <0.05. Full size image The observed evolution towards female patterns of gene expression in the transcriptomes of males and females in monogamous populations indicates that, under the normal polygamous mating system of Drosophila , many genes are constrained from evolving optimal sex-specific expression. The fact that this evolutionary change also occurs in fly heads confirms that the observed feminization is not restricted to sex-limited tissues. Sexually antagonistic selection on gene expression is likely even more extensive than our results indicate because any genes for which males and females experience divergent natural selection, but not sexual selection, are unaffected by our mating system manipulation. The widespread constraints on sexually dimorphic gene expression revealed by our study point to an important role of sexually antagonistic selection in the maintenance of genetic variation, which remains a great puzzle of population genetics [18] . Past work has shown that alleles conferring increased female fitness tend to reduce male fitness on average [19] , [20] and this kind of sexually antagonistic genetic variation is abundant in populations [21] , [22] , [23] . There is evidence that these sexually antagonistic effects on fitness may be mediated by gene expression levels [24] and, consistent with this, our data show that sex-biased genes are current targets of sexually antagonistic selection. In particular, the fact that the expression of these genes evolved in only 65 generations indicates that the ancestral base population must have harboured substantial genetic variation affecting expression despite its long history in a relatively constant laboratory environment. Finally, our study also sheds light on the evolutionary consequences of sexual selection. It has been repeatedly shown that, after removal of sexual selection by enforced monogamy, populations evolve improved reproductive output [9] , [25] , [26] . This has been thought to result mainly from monogamous males evolving to harass females less [25] or to reduce the harmful effects of seminal fluid proteins transferred to females upon mating [27] . Our results point to a complementary, more general explanation. They imply that sexual selection on males combined with constraints on sexually dimorphic gene expression limit the evolution of transcriptomes optimized for female performance, the primary determinant of a population’s reproductive output in species without paternal care. Thus, although sexual selection may facilitate adaptation by promoting good genes [28] , it appears to simultaneously impose a load on populations that negatively affects ecological success. Experimental evolution The fly populations used in the experiments have been described previously [9] . A long-term laboratory population (the IV population) that was initiated from wild D. melanogaster captured in 1975 (ref. 29 ) was subjected to mutagenesis at the outset of the experiment, resulting in the equivalent of 95 generations of spontaneous mutation. After a generation of mass breeding, these flies were subdivided into three monogamous populations in which the opportunity for sexual selection was reduced and three polygamous populations experiencing female choice and male–male competition every generation, with a census size of 200 individuals in each population. In order to enforce monogamy, each generation virgin females were randomly paired with one virgin male each and allowed to spend 2 days mating in interaction vials. In contrast, in polygamous populations groups of five virgin females were combined with groups of five virgin males in vials and also allowed to spend 2 days mating. After 2 days in these interaction vials, males from both treatments were discarded and females from each replicate were placed into two bottles, 50 females per bottle. The mated females spent the next 3 days laying eggs in these bottles before also being discarded. These bottles were the source of the next generation’s flies, which were passed back through the experimental treatment. Whole-fly expression profiling and analysis After 65 generations, the three experimentally evolved monogamous and polygamous populations were all reared in a common garden (the monogamous mating scheme) for one generation and then virgin males and females were collected and held in same sex groups of 10 individuals. After 4 days, total RNA was extracted from whole flies from all of the groups using RNAzol (Molecular Research Center). Double-stranded cDNA was then synthesized using the Invitrogen Superscript II kit, fluorescently labelled and hybridized to Roche Nimblegen 12 × 135 k arrays. There were a total of 12 samples (6 populations × 2 sexes) in the experiment. The arrays were scanned to produce raw signal intensity values for all probes. These values were then preprocessed using the RMA (Robust Multichip Average) algorithm. For analyses of sex-biased gene expression evolution, a gene was considered sex-biased if there was a significant sex effect (false discovery rate of 10%) in the meta-analysis of whole-fly microarray studies (SEBIDA [11] ). Using more restrictive thresholds (for example, a minimum twofold difference in expression between the sexes) does not qualitatively change the results of any of the analyses. The log 2 fold difference between females and males was also obtained from SEBIDA. Change under monogamy for each sex was the average log 2 expression value in monogamy minus the average log 2 expression value in polygamy. Two-sample independent t -tests were used to determine whether the change under monogamy was significantly different in male- or female-biased genes as compared with unbiased genes, which were defined as those with no significant sex effect and a fold difference between the sexes of less than 1.5. For testing genes absent from all sex-limited tissues (male testes and accessory gland, female ovaries and spermatheca), a gene was considered to be absent if it was called present in two or fewer out of the four arrays available for each tissue in the FlyAtlas [12] dataset. Head expression profiling and analysis After 117 generations, the three experimentally evolved monogamous and polygamous populations were all reared in a common garden (the monogamous mating scheme) for one generation, and then virgin males and females from all populations were collected across 4 consecutive days and held in same sex groups of 10 individuals. At 4 days of age, flies were briefly anesthetized between 9:00–11:00 and heads were dissected into liquid nitrogen. Total RNA was extracted from these heads using RNAzol (Molecular Research Center). Libraries were generated using Illumina’s mRNA-Seq preparation kit for the 12 samples (6 populations × 2 sexes) and four lanes, each with all libraries multiplexed, were sequenced on a HiSeq 2500 using single-end chemistry. The reads generated, along with reads for fly heads from the modENCODE project [17] , were mapped first to the D. melanogaster annotated transcriptome using Tophat2 (ref. 30 ). Those that did not map on the transcriptome were then mapped to the genome (BDGP5). The mapped reads were assigned to features of the D. melanogaster transcriptome using HTSeq ( http://www-huber.embl.de/users/anders/HTSeq/ ). This yielded between 34 and 53 million mapped reads assigned uniquely to genomic features (genes) for each sample. Count data were then normalized for library size (genes with at least one normalized read per sample were retained for further analyses) in the DESeq2 package [31] of the BioConductor [32] suite. To obtain a measure of sex-biased gene expression from an independent source, we also ran a generalized linear model on the modENCODE head data with DESeq2 in order to determine which genes’ expression was significantly affected by sex. The resulting list of sex-biased genes, and their estimated magnitude of sex bias, was used in further analyses of evolutionary change in our experimental populations. Change under monogamy for each sex was the average log 2 expression value in monogamy minus the average log 2 expression value in polygamy. Two-sample independent t -tests were used to determine whether the change under monogamy was significantly different in male- and female-biased genes as compared with unbiased genes, which were defined as those with no significant sex effect and a fold difference between the sexes of less than 1.5. Accession Codes : Microarray data have been deposited at the Gene Expression Omnibus (GEO) under the accession code GSE39742 . RNA-Seq data have been deposited at the GEO under the accession code GSE50915 How to cite this article : Hollis, B. et al. Evolution under monogamy feminizes gene expression in Drosophila melanogaster . Nat. Commun. 5:3482 doi: 10.1038/ncomms4482 (2014).